Southern Annular Mode-like changes in southwestern Patagonia at centennial timescales over the last three millennia Late twentieth-century instrumental records reveal a persistent southward shift of the Southern Westerly Winds during austral summer and autumn associated with a positive trend of the Southern Annular Mode (SAM) and contemporaneous with glacial recession, steady increases in atmospheric temperatures and CO 2 concentrations at a global scale. However, despite the clear importance of the SAM in the modern/future climate, very little is known regarding its behaviour during pre-Industrial times. Here we present a stratigraphic record from Lago Cipreses (51°S), southwestern Patagonia, that reveals recurrent ~200-year long dry/warm phases over the last three millennia, which we interpret as positive SAM-like states. These correspond in timing with the Industrial revolution, the Mediaeval Climate Anomaly, the Roman and Late Bronze Age Warm Periods and alternate with cold/wet multi-centennial phases in European palaeoclimate records. We conclude that SAM-like changes at centennial timescales in southwestern Patagonia represent in-phase interhemispheric coupling of palaeoclimate over the last 3,000 years through atmospheric teleconnections. Historical and palaeoclimate records from the North Atlantic and Europe were the first to reveal centennial-scale swings in temperature and precipitation over the last millennia, the most recent of which are referred to as the Medieval Warm Period (also named the Medieval Climate Anomaly, MCA, 0.8–1.1 ka (ka=10 3 cal yr BP (calendar years before present, present=AD 1950)), AD 1350–750) and the Little Ice Age (LIA, 0.1–0.6 ka, AD 1850–1350) [1] . These climatic anomalies occurred during profound land-use changes and before large increases in atmospheric greenhouse gas concentrations associated with the Industrial Revolution. Therefore, studying the timing, structure, magnitude, direction and geographic variability of centennial-scale events such as the MCA and the LIA may help us to understand the causes and consequences of climate change under natural boundary conditions not dissimilar from the modern. More recent studies carried out in the tropics and subtropics have suggested that centennial-scale changes in precipitation regimes have occurred over the last two millennia, with alternations between modes of variability akin to the modern functioning of the El Niño-Southern Oscillation [2] , [3] . Heterogeneities in timing and direction of changes are evident among these low-latitude records, possibly reflecting antiphased response patterns or varying degrees of stationarity of the climate teleconnections among the studied regions. Little is known, however, about centennial-scale changes in temperature and precipitation regimes in the southern extra tropics during the most recent millennia, a vast sector characterized by a strong zonal atmospheric circulation pattern imparted by the Southern Westerly Winds (SWW) [4] . Late twentieth century instrumental and reanalysis data indicate an acceleration and southward shift of the SWW during austral summer and autumn [5] , contemporaneous with a global warming trend, increasing atmospheric CO 2 concentrations and persistently positive phases of the SAM [6] (also known as the Antarctic Oscillation), the main mode of atmospheric variability in the mid- and high-latitudes of the Southern Hemisphere (SH; Supplementary Discussion ). This atmospheric trend has been attributed to human-induced changes in atmospheric chemistry during the twentieth century [7] . The shortness of climate records from the SH, however, impedes appreciation of whether this phenomenon is superimposed on natural, low-frequency climate variability. Modelling and empirical studies have proposed that variations in SWW-driven upwelling over the Southern Ocean (SO) have modulated ocean-atmospheric CO 2 fluxes through degassing of the deep ocean during key climatic transitions, that is, glacial terminations [8] , [9] , millennial-scale shifts during the last glaciation and the Holocene [10] , [11] . Hence, it is of uttermost importance to determine whether the SWW-SO-CO 2 -coupled system holds for the most recent centuries and millennia, as it may constitute a source of positive climate feedback that needs to be fed into numerical simulations of future climate change under various global warming scenarios. Patagonia is a key region to examine variations of the SWW in the middle latitudes of the SH. The amount of precipitation along its western sector exhibits a positive and significant correlation with low-level zonal wind intensity over a broad swath of the southern mid-latitudes [12] ( Fig. 1 ). Climate analyses have also detected a strong positive correlation between SAM and temperature throughout Patagonia (40°–54°S) and a negative correlation with zonal wind intensity and precipitation during summer in Patagonian sectors north of ~50°S ( Supplementary Discussion and Supplementary Figs 1–3 ). The sign of these SAM-related climate anomalies over Patagonia is notably stable between the pre- and post-1979 periods, consistent with the location of the study area well into the southern mid-latitudes, unlike the less stable SAM-related anomalies in subtropical South America [13] ( Supplementary Discussion ). Tree-ring studies along sectors adjacent to the western and eastern flanks of the northern and southern Patagonian Andes detected anomalous growth patterns [14] over the last 600 years, associated with temperature/precipitation anomalies characteristic of the SAM. Moreover, fire-scarred tree data along western Patagonia reveal increased fire activity associated with positive departures of the SAM [15] . 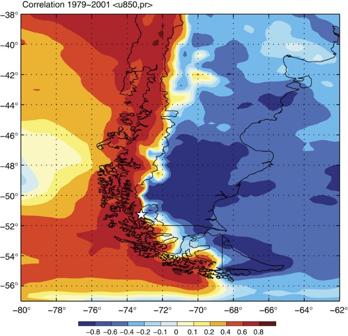Figure 1: Map of the study area and correlation fields between local precipitation and zonal wind speed. We correlated the zonal wind at 850 hPa from a regional climate simulation (PRECIS) forced by ERA40 lateral boundary conditions (see details in ref.4), for the period 1979–2001. The white star indicates the location of Lago Cipreses. Figure 1: Map of the study area and correlation fields between local precipitation and zonal wind speed. We correlated the zonal wind at 850 hPa from a regional climate simulation (PRECIS) forced by ERA40 lateral boundary conditions (see details in ref. 4 ), for the period 1979–2001. The white star indicates the location of Lago Cipreses. Full size image Vegetation composition and distribution in southwestern Patagonia are highly dependent on precipitation delivered by atmospheric disturbances embedded in the SWW. The lowland vegetation of southwestern Patagonia (>48°S) includes Magellanic forest communities, dominated by the evergreen Nothofagus betuloides (Magellanic beech) along with the cold-resistant conifers Pilgerodendron uviferum, Podocarpus nubigena and other hygrophilous trees ( Drimys winteri , Tepualia stipularis ) that intermingle with Magellanic Moorlands in the wettest sectors (2,000–6,000 mm year −1 ) adjacent to the Pacific coast [16] . The winter-deciduous Nothofagus pumilio is most abundant in lowland forests located downwind (eastward) in less humid areas (~750 mm year −1 ), intermingling with Nothofagus Antarctica -dominated woodlands in drier sectors (~450 mm year −1 ) adjacent to the forest-steppe ecotone. The shrubs Escallonia serrata, Berberis ilicifolia and Embothrium coccineum occur in the margins of N. betuloides- or N. pumilio -dominated forests, and the ferns Blechnum penna-marina , Hymenophyllum spp. are abundant under relatively open canopy conditions or tree-fall gaps. Deciduous forests and woodlands transition into the Patagonian steppe east of the Andes in response to a strong rainshadow induced by the abrupt relief. The composition and distribution of this transition is dependent on the amount of precipitation of westerly origin that spills eastward over the cordillera. Meteorological data from Torres del Paine National Park (51°S), an area located in the forest-steppe ecotone of southwestern Patagonia, exhibit a strong positive correlation between local precipitation and zonal wind intensity [17] ; the strength of this correlation diminishes and turns negative in stations located towards the Atlantic coast [4] . Hence, hydroclimate inferences based on palaeovegetation, past lake level changes and palaeofire-regime shifts from the western sectors of southern Patagonia constitute a valuable source of information for reconstructing past variations of the SWW and SAM. Here we present palynological and fire history data from sediment cores collected from Lago Cipreses (LC), a small closed-basin lake located in the Magallanes region of southern Chile (51°S), to characterize centennial-scale changes in the SWW during the last three millennia akin to the modern functioning of SAM. Vegetation and fire history LC is surrounded by mixed evergreen-deciduous Magellanic forests that have experienced relatively minor disturbance since the arrival of Europeans, owing to the inaccessibility of the area and the natural fire break established by Lago Toro. In contrast, more accessible areas located 20–30 km north (Torres del Paine National Park) and south (Puerto Natales) have witnessed large-scale disturbance by fire, logging and livestock grazing since local European settlement starting in AD 1870 (ref. 18 ). We retrieved sediment cores from LC showing undisturbed, continuous pelagic sedimentation since ~15 ka ( Supplementary Discussion , Supplementary Figs 4–6 ). The pollen and charcoal records show dominance of Nothofagus along with the hygrophilous conifers Pilgerodendron uviferum, Podocarpus nubigena and traces of Drimys winteri since 3 ka ( Fig. 2 , Supplementary Fig. 7 ), which we interpret as local dominance of Magellanic forests with varying degrees of openness in response to environmental change. Over this interval, we detect five intervals (CC1 (CC=Cipreses cycle): AD 1890–present, CC2: 0.8–1.1, CC3: 1.4–1.55, CC4: 1.8–2.1 and CC5: 2.7–2.9 ka) during which the abundance of Nothofagus declined and reached values between 65 and 85%, accompanied by increases in herbs, ferns and macroscopic charcoal, all indicative of fragmentations/discontinuities in the forest canopy, proliferation of understory shrubs/herbs and enhanced fire activity. The macrophyte Cyperaceae covaries (1–7%) with the terrestrial herbs suggesting that littoral vegetation was able to expand towards deeper sectors of the lake repeated times in response to lower stands ( Fig. 2 , Supplementary Fig. 7 ). We note that Escallonia and the siliciclastic density data display nearly identical fluctuations in phase with the aquatic vegetation changes described above, which we interpret as colonization of Escallonia shrublands on the substrates exposed by lake level lowering, increased runoff and erosion associated with vegetation clearings driven by local fires. Each CC is followed by a rise in arboreal pollen reaching maxima between 85 and 95%, decrease in aquatic macrophytes and decline in charcoal, suggesting re-establishment of closed-canopy forests, relatively deep lake conditions and muted fire activity. CC3 and CC4 feature the lowest magnitude of Non-Arboreal Pollen (NAP) rise, followed by CC2, then CC5 and CC1 with the fastest, largest-magnitude increase on record. We note a rapid Nothofagus increase that reached peak abundance between 0.55 and 0.65 ka and declined ~8% gradually until AD 1890, contemporaneous with a sustained rise in P. uviferum of similar magnitude. Both hygrophilous trees decline rapidly at AD 1890 concomitant with an abrupt increase in herbs and shrubs, including the appearance of the European weed Rumex acetosella , along with a conspicuous rise in macroscopic charcoal (CC1; Supplementary Discussion , Supplementary Figs 7–10 ). 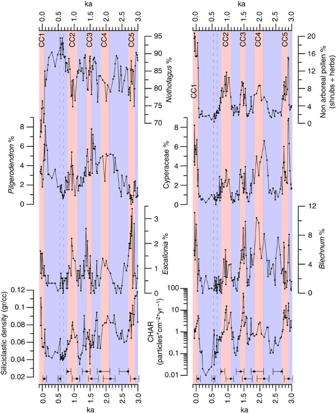Figure 2: Summary of the Lago Cipreses record. We emphasize the timing of dry/warm phases (red vertical rectangles) that alternate with cold/humid phases (blue vertical rectangles). The dashed vertical rectangle indicates the timing of the highest abundance ofNothofagusduring the most recent hyperhumid anomaly. The numbered labels indicate the dry/warm events recorded in the Lago Cipreses record (CC: Cipreses Cycle), the solid black circles in the bottom of the figures indicate the median probability age for the transitions identified in this record, the error bars define the 95% confidence interval associated to these transitions according to a Bayesian age model. Figure 2: Summary of the Lago Cipreses record. We emphasize the timing of dry/warm phases (red vertical rectangles) that alternate with cold/humid phases (blue vertical rectangles). The dashed vertical rectangle indicates the timing of the highest abundance of Nothofagus during the most recent hyperhumid anomaly. The numbered labels indicate the dry/warm events recorded in the Lago Cipreses record (CC: Cipreses Cycle), the solid black circles in the bottom of the figures indicate the median probability age for the transitions identified in this record, the error bars define the 95% confidence interval associated to these transitions according to a Bayesian age model. Full size image Palaeoenvironmental interpretation Taken together, the pollen, charcoal and sedimentary records from LC suggest the occurrence of ~200 year-long dry/warm phases alternating with wet/cold intervals during the last 3,000 years in southwestern Patagonia. Given that precipitation in this sector is derived exclusively from the SWW and that local precipitation and summer temperature are positively/negatively correlated with zonal wind velocity, respectively, we infer secular changes in zonal SWW strength over the study area. The character and direction of these changes suggest large-scale shifts in mid- and high-latitude atmospheric circulation similar to the modern functioning of SAM in Patagonian sectors north of ~50°S during austral summer and autumn, with negative centennial-scale anomalies in precipitation regime and positive air temperature anomalies (positive SAM-like) responsible for intensified fire activity, forest fragmentation, erosion and lake-level lowering. In contrast, we ascribe muted fire activity, lake-level rises and establishment of closed-canopy Magellanic forests to positive centennial-scale anomalies in precipitation and negative temperature anomalies (negative SAM-like). The most recent of these dry/warm phases (CC1) has been in effect since AD 1890 and corresponds in timing with the Industrial Revolution, a persistent southward shift of the SWW during austral summer and a persistent trend towards positive SAM revealed by instrumental records since the mid-twentieth century ( Fig. 3 ). 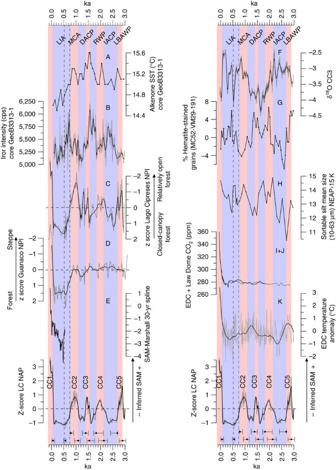Figure 3: Intersite comparisons. We compare the standardized Lago Cipreses Non Arboreal Pollen curve (LC NAP; bottom curves) with the alkenone24(A) and Fe intensity data25(B) from core GeoB3313-1, the standardizedNothofagus/Poaceae Indeces (NPI) from LC (C) and Lago Guanaco19(D), a tree-ring-based reconstruction of SAM14(E), a δ18O speleothem record from Northwestern Ireland28(F), the hematite-stained grain record from North Atlantic cores MC52-VM29-191 (ref.26;G), the sortable silt record from North Atlantic core NEAP-15K27(H), atmospheric CO2records32,33from EDC (I) and Law Dome (J) ice cores, and the temperature anomaly record from EDC31(K). Also shown are the recognized palaeoclimate anomalies from Europe: Little Ice Age (LIA), Medieval Climate Anomaly (MCA), Dark Ages Cold Period (DACP), Iron Age Cold Period (IACP), Late Bronze Age Warm Period (LBAWP). The oblique and partly overlapping acronymns represent uncertainties and/or geographic heterogeneities for their exact onset and duration. The red and blue vertical rectangles represent the warm/dry and cold/wet phases identified in the Lago Cipreses record, respectively. The dashed vertical rectangle indicates the timing of the highest abundance ofNothofagusduring the most recent hyperhumid anomaly. Figure 3: Intersite comparisons. We compare the standardized Lago Cipreses Non Arboreal Pollen curve (LC NAP; bottom curves) with the alkenone [24] (A) and Fe intensity data [25] (B) from core GeoB3313-1, the standardized Nothofagus /Poaceae Indeces (NPI) from LC (C) and Lago Guanaco [19] (D), a tree-ring-based reconstruction of SAM [14] (E), a δ 18 O speleothem record from Northwestern Ireland [28] (F), the hematite-stained grain record from North Atlantic cores MC52-VM29-191 (ref. 26; G), the sortable silt record from North Atlantic core NEAP-15K [27] (H), atmospheric CO 2 records [32] , [33] from EDC (I) and Law Dome (J) ice cores, and the temperature anomaly record from EDC [31] (K). Also shown are the recognized palaeoclimate anomalies from Europe: Little Ice Age (LIA), Medieval Climate Anomaly (MCA), Dark Ages Cold Period (DACP), Iron Age Cold Period (IACP), Late Bronze Age Warm Period (LBAWP). The oblique and partly overlapping acronymns represent uncertainties and/or geographic heterogeneities for their exact onset and duration. The red and blue vertical rectangles represent the warm/dry and cold/wet phases identified in the Lago Cipreses record, respectively. The dashed vertical rectangle indicates the timing of the highest abundance of Nothofagus during the most recent hyperhumid anomaly. Full size image We standardized the LC NAP curve to the mean of the last three millennia to summarize the major trends in the LC record and facilitate comparisons with other studies. Positive anomalies in this parameter are interpreted as warm/dry intervals analogue to positive SAM-like states; negative anomalies correspond to cool humid/hyperhumid intervals and are interpreted as negative SAM-like states ( Fig. 3 ). Comparison with the Nothofagus /Poaceae Index from Lago Guanaco (LG) [19] , a palecoecological site located ~30 km downwind from LC in a sector adjacent to the modern forest-steppe ecotone, reveals large-magnitude shifts associated with CC5, the hyperhumid interval between AD 1890-0.65 ka and CC1 ( Fig. 3 ). These shifts reflect major physiognomic changes in the vegetation near LG from a graminoid steppe to a Nothofagus scrubland at 2.8 ka, followed by forest expansion at ~0.8 ka and rapid deforestation at AD 1890 driven by intense European disturbance. The relatively minor or muted changes between approximately 0.8 and 2.8 ka might reflect resilience of Nothofagus scrublands located near the forest-steppe ecotone to natural climate/disturbance variability under intermediate levels of precipitation. In contrast, the continuity of the forest canopy revealed by the LC Nothofagus /Poaceae Index parameter shows high sensitivity to the CCs and intervening humid phases, illustrating the capacity of forest vegetation to recover its original condition following natural climatic/disturbance disruptions at centennial timescales. Both the LC and LG records compare reasonably well with a recent reconstruction of SAM that spans the last 600 years [14] based on an extensive network of tree-ring chronologies from Tasmania, New Zealand and sectors of Patagonia located east and west of the Andes, north and south of LC. The hyperhumid phase dated in LC between AD 1890 and 0.65 ka is contemporaneous with strongly negative anomalies in tree-ring inferred SAM ( Fig. 3 , Supplementary Fig. 9 ) and the maximum extent of multiple alpine glaciers in Patagonia [20] and the southern Alps of New Zealand [21] . This was followed by an abrupt onset of warm/dry conditions and intense fire activity at the onset of CC1 (AD 1890, ±2σ: 1933–1818) contemporaneous with a rising trend in tree-ring-based temperature reconstructions from northern and southern Patagonia [22] , and predate a rapid increase in tree-ring-reconstructed SAM at AD 1950. The tree-ring reconstruction and time-series analysis of weather station data published by Villalba et al. [14] , along with our stratigraphic record from LC and regional climate analysis, indicate that carefully selected sites from sensitive sectors throughout Patagonia are capable of monitoring hemispheric-wide modes of variability such as SAM, despite the complex relief and climatic heterogeneity stressed in a recent study [23] . We now compare the timing and structure of palaeoclimate changes observed in LC with palaeoclimate records from the SE Pacific and North Atlantic/European regions. Figure 3 shows the alkenone [24] and Fe intensity data [25] from core GeoB3313-1, obtained from the Chilean continental slope (~41°S) and interpreted as sea surface temperature and amount of precipitation delivered by the SWW in northwestern Patagonia, respectively. We observe an apparent match between the LC NAP and the alkenone record and a variable relationship with the Fe intensity record, which might represent an in-phase, antiphase or out-of-phase precipitation pattern between northwestern and the LC record, depending on the interpretation of the Fe intensity data ( Supplementary Discussion ). We also compare our results with proxies of ice-rafting [26] , intensity of Atlantic Meridional Overturning Circulation (AMOC) [27] preserved in North Atlantic sediment cores and air temperature change recorded in a speleothem from Crag Cave in SW Ireland [28] since 3 ka. We note partial convergence among these North Atlantic records and the European palaeoclimate chronology, suggesting regional heterogeneities at centennial timescales or differences in chronologic precision/accuracy/sensitivity of the selected records. Acknowledging these sources of error, we observe that CC1, CC2, CC4 and CC5 were quasi-contemporaneous with the twentieth century industrial warming, the Mediaeval (=MCA), Roman and Late Bronze Age Warm Periods, respectively ( Fig. 3 , Supplementary Discussion ). The intervening hyperhumid (AD 1890–0.8 ka) and humid (1.1–1.8, 2.1–2.7 ka) phases overlap in timing with the LIA, the Dark Ages (DACP) and Iron Age Cold Periods, respectively. The 1.1–1.8 ka cold/wet interval is punctuated a ~150-year long variable phase in the LC record (CC3), which does not correlate with any distinct recognized palaeoclimate event in the NH, but was contemporaneous with a strongly variable warm pulse in the speleothem record shown in Fig. 3 and, within radiocarbon dating errors, a trough in the ice-rafted detritus data and a prominent peak in the sortable silt record ( Supplementary Discussion ). Our results suggest that centennial-scale changes in SAM shared a common structure and timing, within dating uncertainties, with palaeoclimate records from the NH over the last 3000 years. The mechanism(s) governing this interhemispheric symmetry are currently unknown; if replicated by additional high-resolution precisely dated records, this correspondence would imply that palaeoclimate in the northern and southern mid-latitudes were linked through a mechanism residing in the atmosphere, possibly through poleward expansions of Hadley cell circulation [29] , solar variability [26] or, alternatively, through a closely tuned interhemispheric SWW-SO-AMOC-coupled system [30] . Centennial-scale warm phases in the EPICA Dome C (EDC) ice core from Antarctica [31] lag behind CC3 and CC5 but coincided in timing during CC1 ( Fig. 3 ), aspect that might reflect non-stationarities in the temperature change correlation between eastern Antarctica and SAM. The atmospheric CO 2 record from Antarctic ice cores [32] , [33] shows erratic, low-magnitude variations before the Industrial Revolution that bear no clear relationship with the LC record and EDC temperatures, suggesting that pre-industrial changes in the position/strength of the SWW and temperature change in eastern Antarctica since 3 ka were not associated with any salient shifts in the atmospheric CO 2 content at centennial timescales. Quite a different situation occurs during the Industrial Revolution (CC1), a time when a prominent CO 2 rise correlates with a sustained rise in Antarctic and global temperatures and a positive trend in instrumental, tree-ring and our estimate of palaeo SAM activity. The LC record suggests that the current trend towards positive SAM resembles pre-industrial oscillations that have taken place repeated times over the last three millennia in the southern mid-latitudes. The amplitude of the modern excursion, however, is unprecedented, suggesting that direct (vegetation disturbance) or indirect (atmospheric circulation changes) human perturbations have influenced vegetation change in the LC record since the late nineteeth century. Because recent studies have proposed that the contemporary trend towards positive SAM is largely driven by stratospheric ozone depletion and, secondarily, to increased greenhouse gases [7] , we propose that a juxtaposition of anthropogenic and natural forcing of the SH climate since the nineteeth century has forced an austral summer poleward shift and year-round intensification of the SWW into sensitive sectors of the SO where intense degassing of CO 2 -enriched deep waters currently takes place. This scenario raises the disturbing possibility that intensified SWW-driven upwelling in the SO could lock enhanced release of greenhouse gases from the deep ocean, providing an additional source of positive radiative forcing of future global climate in an already warming world. Stratigraphy LC (51.285025°S, 72.853494°W, 110 m.a.s.l.) is a small closed-basin lake located on an ice-scoured bedrock depression over a mountainous terrain near the southwestern sector of Lago Toro (120 m.a.s.l.). Here we obtained three overlapping sediment cores from an anchored raft equipped with a 10-cm wide aluminum casing, using a 5-cm diameter Wright piston corer and a sediment–water interface piston corer with a 7.5-cm diameter Plexiglas chamber. The cores were taken from the deepest sector of the lake following a bathymetric survey with a sonar. We retrieved overlapping Wright cores PS0710A (287 cm long) and PS0710B (197 cm long), along with the sediment–water interface core PS07SC1 (83 cm long). Correlation between cores was facilitated by results of the loss-on-ignition analysis and the presence of a 3-cm thick tephra at depth 77–80 cm in cores PS0710A and PS07SC1 ( Supplementary Fig. 4 ). The stratigraphy of the cores was characterized by lithological descriptions, digital X-radiographs and loss-on-ignition analysis following overnight drying at 105 °C. We performed sequential burns at 550 and 925 °C for 2 and 4 h, respectively, to quantify the organic, carbonate and siliciclastic content of the sediments [34] , [35] . Identification and correlation of tephras with known eruptions of specific source volcanoes in the region [34] were based on petrology and trace-element chemistry determined by inductively coupled plasma mass spectrometry (ICP-MS) analysis. The record shown in this paper includes the upper 121 cm of the spliced stratigraphy, which consists of silty organic lake mud devoid of carbonates, with a mean organic content of 30% ( Supplementary Fig. 4 ). Geochemical analysis indicates that the tephra was derived from Volcán Reclús (C. Stern, personnel communication). Chronology The chronology of the sediment cores is controlled by 210 Pb and AMS radiocarbon dates ( Supplementary Figs 4 and 5 ) obtained from bulk 1-cm thick sections along the cores. All radiocarbon dates were converted to cal yr BP using the IntCal09 calibration curve included in the CALIB 6.0 software [36] . Based on the radiocarbon data we developed a Bayesian age model ( Supplementary Fig. 6 ) to assign interpolated calendar ages to the levels analysed ( Supplementary Fig. 7 ) using the Bacon package [37] for R. We used the median probability age calculated for each level and specified the 95% confidence intervals for each major transition in the LC record. Supplementary Table 3 summarizes the median age probability and associated confidence intervals for the onset and termination of each CC in cal yr BP and AD/BC timescales. The 210 Pb concentrations were interpreted using the constant rate of supply model of 210 Pb accumulation ( Supplementary Table 1 and Supplementary Fig. 5 ). In addition, we obtained three AMS radiocarbon dates from core PS0710SC1 and four additional from core PS0710A ( Supplementary Table 2 ). The age model takes into account the 210 Pb and AMS radiocarbon dates and the instantaneous deposition of the ~1900 cal yr BP-old tephra. The age model has a median deposition time of 20 years cm −1 (25.8±20.3 year cm −1 (mean±1σ), minimum: 2.1 year cm −1 at 18 cm, maximum: 98.8 year cm −1 at 14 cm). The chronology of the Reclús tephra at depth 77–80 cm is constrained by the date of sample CAMS-149318 (1.765±30 14 C yr BP, median probability: 1,620 cal yr BP) and constitutes a close minimum limiting age for this event. This date shows good agreement with radiocarbon dates obtained from Pantano Margarita and LG [19] , sites having depositional settings similar to LC, which yielded a close maximum limiting weighted mean age of 2,000±17 14 C yr BP (1,950 cal yr BP). Palynology and charcoal analysis We processed 2 cc sediment samples for pollen analysis using standard techniques that include KOH deffloculation, concentrated HF treatment and acetolysis [38] . We added Lycopodium spore tablets to the sediment samples to allow calculation of pollen and charcoal concentration and accumulation rates. The concentrates were mounted on glass slides in a silicon oil (2,000 cs) medium and analysed at × 400 and × 1,000 magnification using an Olympus CX31 stereomicroscope. The record shown in this paper consists of 118 palynological levels spanning the last 3,000 years with a median time resolution of 20 years between levels ( Supplementary Fig. 7 ). We counted the pollen and spore content of these samples considering a mean of 586 grains of terrestrial origin per level (minimum: 118, maximum: 1,300), and calculated their percent abundance as a function of this pollen sum. In the case of aquatic plants and ferns, we calculated percentages in reference to sums that included all pollen grains (terrestrial and aquatic) and spores, respectively. Variations in the abundance of these main components are independent considering that their percent abundances were calculated from different, independent sums. The palynological results are shown as percentage data in Supplementary Figs 7–9 and depict variations in the most abundant and informative pollen taxa. Taxa are arranged in terms of terrestrial (arboreal+non arboreal) and aquatic pollen, along with fern spores. We analysed the macroscopic charcoal content of 2-cc sediment samples taken at contiguous 1-cm thick intervals using the methodology described by Whitlock and Anderson [39] , which includes deflocculating with 10% KOH and sieving through 106- and 212-μm mesh screens. We counted charcoal particles in each size class under a Zeiss KL1500 LCD stereomicroscope at × 50–100 magnification. The abundance of macroscopic charcoal particles is expressed as charcoal accumulation rate in linear or logarithmic scale ( Supplementary Fig. 10 ). How to cite this article: Moreno, P. I. et al. Southern Annular Mode-like changes in southwestern Patagonia at centennial timescales over the last three millennia. Nat. Commun. 5:4375 doi: 10.1038/ncomms5375 (2014).